Increased atrial arrhythmia susceptibility induced by intense endurance exercise in mice requires TNFα Atrial fibrillation (AF) is the most common supraventricular arrhythmia that, for unknown reasons, is linked to intense endurance exercise. Our studies reveal that 6 weeks of swimming or treadmill exercise improves heart pump function and reduces heart-rates. Exercise also increases vulnerability to AF in association with inflammation, fibrosis, increased vagal tone, slowed conduction velocity, prolonged cardiomyocyte action potentials and RyR2 phosphorylation (CamKII-dependent S2814) in the atria, without corresponding alterations in the ventricles. Microarray results suggest the involvement of the inflammatory cytokine, TNFα, in exercised-induced atrial remodelling. Accordingly, exercise induces TNFα-dependent activation of both NFκB and p38MAPK, while TNFα inhibition (with etanercept), TNFα gene ablation, or p38 inhibition, prevents atrial structural remodelling and AF vulnerability in response to exercise, without affecting the beneficial physiological changes. Our results identify TNFα as a key factor in the pathology of intense exercise-induced AF. Atrial fibrillation (AF) is the most common arrhythmia that is associated with ageing as well as hypertension, structural heart disease, hyperthyroidism and several other cardiovascular conditions [1] . Although exercise is known to provide enormous health benefits particularly by improving disease outcomes in cardiovascular patients [2] , it is now clear that high intensity endurance sports increase AF susceptibility in the absence of underlying cardiovascular disease [3] , [4] , [5] , [6] . The basis for the association between intense exercise and AF is poorly understood. AF is generally associated with atrial remodelling often characterized by increased parasympathetic nerve activity (PNA) [7] , atrial enlargement [8] , fibrosis [9] and inflammation [10] . A hallmark of endurance athletes is heart rate slowing due to elevated parasympathetic tone [11] and atrial hypertrophy [12] both risk factors for AF. Intense physical activity also elevates inflammatory factors such as CRP [13] and TNFα [14] , which can be activated by atrial stretch following elevated atrial pressures (~35 mm Hg) as occurs during intense exercise [15] . Indeed, although expression of TNFα was originally thought to originate primarily from macrophages [16] , other cells such as cardiac myocytes synthesize TNFα in response to myocardial stretch [17] , [18] and elevated cardiac TNFα induces atrial fibrosis, myocardial hypertrophy and AF [19] . In this study we show that intense endurance exercise (involving swimming or treadmill running for 6 weeks) increases susceptibility to AF in mice and is associated with macrophage infiltration and fibrosis. This exercise-induced atrial remodelling is prevented by treatment with the TNFα inhibitor (etanercept) and is not seen in mice lacking TNFα gene. Physiological cardiac remodelling in exercised mice Although the primary purpose of our studies was to assess the link between endurance exercise and cardiac arrhythmias, we began by characterizing our exercised mice. Six-week-old male mice were selected for swimming and treadmill running exercise at levels that exceeded 70% of the VO 2 max for the entire duration of their training protocols ( Supplementary Fig. 1A ), which is similar to levels targeted by elite athlete training programmes [20] . All the mice were trained for 6 weeks (unless otherwise stated), and all the exercised mice were used in subsequent analysis (See Methods). As expected from previous studies examining endurance athletes [11] , heart rates estimated using telemetry ECG measurements declined (swim P =0.009, treadmill P =0.03, one-way ANOVA) progressively after initiating exercise ( Fig. 1 & Supplementary Fig. 1C ). The heart-rate differences ( P <0.01, two-way ANOVA) resulting from exercise were eliminated by blocking the autonomic nervous system (via combined atropine and propranolol treatment, Fig. 1c ). In addition, there were no differences ( P =0.7, Student’s t -test) in beating rates of isolated atria (which lack autonomic nerve inputs) between exercise and sedentary groups ( Fig. 1d ). These results support the conclusion that the exercise-induced reductions in heart rate arise primarily from differences in autonomic nerve activity, as typically seen in athletes [11] . 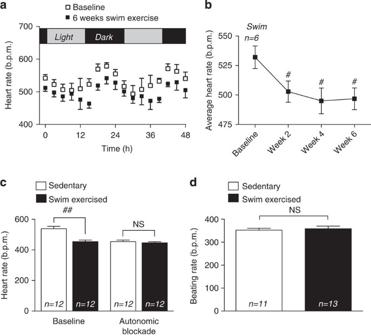Figure 1: Exercise-induced heart rate reductions is mediated by the autonomic nervous system. (a) Three-hour means of HR acquired over a 48-h period in mice implanted with telemetery ECG, at baseline and after 6 weeks of swimming exercise, illustrate preserved circadian oscillations of HR and reductions in HR at all time points over the 48-h period as a result of exercise. Bar indicates day-night cycles. (b) Averaged heart rates (over 48 h) measured using telemetric ECGs in mice exercised by swimming show significant reductions in HR after 4 weeks of swimming exercise. (c) Heart rates derived from surface ECGs in anesthetized mice before and after autonomic blockade using atropine & propranolol. Administration of atropine and propranolol eliminated heart rate differences between 6-week exercised and sedentary mice. (d) To further assess the role of autonomic nerve input on exercise-induced HR reductions, atria were isolated and completely denervated. Field recordings of spontaneously beating atria were used to calculate beating rate. Thenvalues in bars indicate number of mice used. Beating rates of denervated atriaex vivodid not differ between sedentary and 6-week exercised mice. Data presented as mean± s.e.m.,#P<0.05 when compared with baseline using repeated measure one-way ANOVA with Dunnett’s multiple comparison test.##P<0.05 when compared with baseline using repeated measure two-way ANOVA with Sidak’s multiple comparison test. NS, not significant. Ventricles of exercised mice also underwent physiological remodelling, as in athletes [21] , characterized by left ventricular chamber enlargement ( P =0.04, Student’s t -test) and enhanced ventricular contractility at rest ( P =0.002, Student's t -test) as well as following intraperitoneal injection of 1.5 μg g −1 dobutamine ( P =0.006, Student’s t -test), as detailed in Table 1 , Supplementary Tables 1–3 and Supplementary Fig. 2 . Figure 1: Exercise-induced heart rate reductions is mediated by the autonomic nervous system. ( a ) Three-hour means of HR acquired over a 48-h period in mice implanted with telemetery ECG, at baseline and after 6 weeks of swimming exercise, illustrate preserved circadian oscillations of HR and reductions in HR at all time points over the 48-h period as a result of exercise. Bar indicates day-night cycles. ( b ) Averaged heart rates (over 48 h) measured using telemetric ECGs in mice exercised by swimming show significant reductions in HR after 4 weeks of swimming exercise. ( c ) Heart rates derived from surface ECGs in anesthetized mice before and after autonomic blockade using atropine & propranolol. Administration of atropine and propranolol eliminated heart rate differences between 6-week exercised and sedentary mice. ( d ) To further assess the role of autonomic nerve input on exercise-induced HR reductions, atria were isolated and completely denervated. Field recordings of spontaneously beating atria were used to calculate beating rate. The n values in bars indicate number of mice used. Beating rates of denervated atria ex vivo did not differ between sedentary and 6-week exercised mice. Data presented as mean± s.e.m., # P <0.05 when compared with baseline using repeated measure one-way ANOVA with Dunnett’s multiple comparison test. ## P <0.05 when compared with baseline using repeated measure two-way ANOVA with Sidak’s multiple comparison test. NS, not significant. Full size image Table 1 Physical parameters of mice exercised for 6 weeks. Full size table Increased vulnerability to atrial arrhythmias in exercised mice As documented in Fig. 2 (also Supplementary Figs 4–6 ), programmed electrical stimulations ( Supplementary Fig. 4 ) revealed that sustained atrial, but not ventricular, arrhythmias (i.e., bouts of rapid electrical activity lasting >10 s) were induced more frequently in mice undergoing swimming (16/43, P <0.01, χ 2 -test) and treadmill (14/29, P <0.01, χ 2 -test) exercise compared with sedentary controls (1/41). These results establish clear differential effects of exercise on atria versus ventricles. No spontaneous atrial arrhythmias were observed, however, in telemetry ECG recordings of swim or treadmill exercised mice during the 6-week training period. To characterize the AF events, electrical activity of isolated atria was determined (using Di-4-ANEPPS) following programmed field stimulation. As summarized in Fig. 2e,f (and Supplementary Fig. 5C ), AF also occurred ( P <0.03, χ 2 -test) in isolated atria from swimming (5/13) and running (7/16) mice versus sedentary mice (1/15). Analysis of AF events in isolated atria ( Supplementary Figs 7 and 8 ) revealed dynamic and complex ECG electrical activity characterized by transient periodic rapid focal activity and re-entry circuits accompanied by variable conduction block, as described in humans and other animal models [1] , [22] . 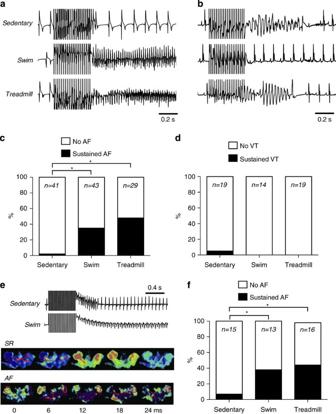Figure 2: Increased vulnerability to atrial but not ventricular arrhythmias in exercised animals. Vulnerability to atrial or ventricular arrhythmias was assessedin vivousing an intracardiac catheter placed in the right ventricle. Representative intracardiac bipolar electrograms showing induction of atrial arrhythmias (a) as well as surface electrogram recordings in the lead II configuration showing induction of ventricular tachyarrhythmias (VT;b) from sedentary, swimming and treadmill exercised mice. The percentage of animals with sustained (>10 s) atrial (c) but not VT (d) is increased significantly by exercise. (e) A typical representative AF event initiated in isolated (denervated) atria by rapid stimulation recorded using field recording (top) and optical mapping images of atria loaded with a voltage sensitive dye during sinus rhythm (SR) and during AF (bottom). Note the disorganized wave propagation during an AF episode. Red arrows indicate the wave-front pathway. (f) Percentage of isolated atria from each group showing sustained AF episodes (>10 s). Thenvalue for each group is indicated on bar graphs and present number of mice.χ2-test *P<0.05. Figure 2: Increased vulnerability to atrial but not ventricular arrhythmias in exercised animals. Vulnerability to atrial or ventricular arrhythmias was assessed in vivo using an intracardiac catheter placed in the right ventricle. Representative intracardiac bipolar electrograms showing induction of atrial arrhythmias ( a ) as well as surface electrogram recordings in the lead II configuration showing induction of ventricular tachyarrhythmias (VT; b ) from sedentary, swimming and treadmill exercised mice. The percentage of animals with sustained (>10 s) atrial ( c ) but not VT ( d ) is increased significantly by exercise. ( e ) A typical representative AF event initiated in isolated (denervated) atria by rapid stimulation recorded using field recording (top) and optical mapping images of atria loaded with a voltage sensitive dye during sinus rhythm (SR) and during AF (bottom). Note the disorganized wave propagation during an AF episode. Red arrows indicate the wave-front pathway. ( f ) Percentage of isolated atria from each group showing sustained AF episodes (>10 s). The n value for each group is indicated on bar graphs and present number of mice. χ 2 -test * P <0.05. Full size image Autonomic and electrical remodelling in atria of exercised mice Candidate mechanisms for increased AF vulnerability with exercise include abbreviated action potential durations (APD) [23] and increased APD heterogeneity [24] both of which can occur with activation of muscarinic K + currents (I K,Ach ) following parasympathetic nerve activity (PNA) [25] . Consistent with a role for elevated PNA, exercised mice showed larger HR responses to atropine than sedentary controls ( Fig. 3a ), and the heart rate variability component, which is associated with PNA [11] , was elevated in exercised mice ( Fig. 3b , Supplementary Fig. 9 ). Furthermore, blockade of the PNA with atropine caused the effective refractory period (ERP) to be longer in exercised mice compared with sedentary ( Fig. 3c ), despite the lack of ERP differences in the absence of drug ( Supplementary Table 4 ). 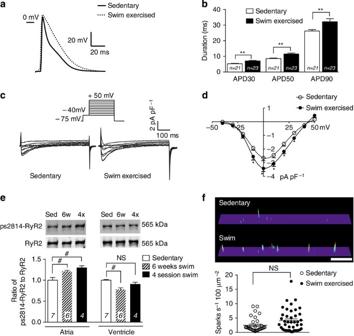Figure 4: Increased action potential durations and ICain the atria of exercised mice. (a) Representative averaged action potentials recorded using sharp microelectrode in isolatedex vivoatria from sedentary and swimming exercised mice. (b) Six weeks of exercise increased the average time to 30, 50 and 90% repolarization (APD30, APD50 and APD90) of left atrial myocytes.N=21/6 mice for sedentary,n=23/6 mice for exercise. (c) Representative ICarecordings in left atrial myocytes using whole-cell patch-clamp. (d) ICaI-V curves in left atrial myocytes showing increase in ICain 6-week exercised mice;n=14 myocytes/3 mice for exercised andn=12/3 mice for sedentary. (e) Increased RyR2 phosphorylation at S2814 in atria of 6 week (6w) and four session (4x) swim exercised mice as compared with sedentary (Sed) mice. Please note the reduction in RyR2 phosphorylation in the ventricles of 6-week swim exercised mice. Thenvalues indicated on bar graph and represent number of mice. (f) Ca2+spark activity in the atria of swim and sedentary exercised mice with representative spark activity shown in top panel;n=35/3 mice for sedentary,n=42/3 mice for exercise. Scale bar, 200 ms. Data presented as mean±s.e.m. *P<0.05 compared with sedentary at the same membrane potential using Student’st-test. **P<0.01 compared with sedentary using Student’st-test.#P<0.05 using one-way ANOVA. However, although atropine prolonged ERPs, it could not entirely prevent AF in exercised mice ( Fig. 3d ). These effects of PNA blockade on ERP and AF in exercised mice are consistent with the longer action potential durations (APDs) in isolated exercised atria and cardiomyocytes ( Fig. 4a,b ), which were associated with increased L-type Ca 2+ currents ( Fig. 4c,d ) without changes in voltage-gated K + currents or I K,Ach (peak amplitude, desensitization or deactivation) measured in atrial cardiomyocytes from exercised mice ( Supplementary Fig. 10 ). As altered RyR2 function has been linked to AF in humans [26] , [27] and mice [28] , pathological cardiac remodelling [29] , and elevated oxidative stress [30] with exercise [31] , RyR2 phosphorylation and oxidation levels were measured. We found increased ( P <0.05, One-way ANOVA) RyR2 phosphorylation at S2814 in the atria from mice after 6 weeks of swimming or after only four sessions of swimming ( Fig. 4e ). Interestingly, the level of phosphorylation at S2814 in the ventricles was significantly decreased in mice after 6 weeks of swimming. In contrast, no differences in RyR2 oxidation, or RyR2 phosphorylation at position S2808 (PKA-dependent) or CaMKII phosphorylation at T287 were detected between the groups ( Supplementary Fig. 11 ). In addition, no change in the expression level of RyR2 or CaMKII was seen between the groups ( Supplementary Fig. 11 ). Elevated RyR2 phosphorylation at 2814 correlated with trends towards increased Ca 2+ spark activity ( P =0.06, Fig. 4f , Student’s t -test) as well as Ca 2+ transient amplitudes ( P =0.06, Supplementary Fig. 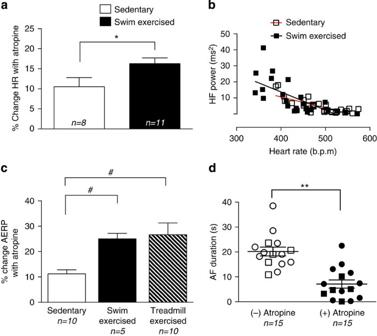11 , Student’s t -test) with no change in Ca 2+ transient decay rates in swimming exercised atrial myocytes as compared with sedentary mice. Figure 3: Effects of atropine on AF susceptibility in exercised mice. (a) Administration of 2 mg kg−1atropine had a larger effect on heart rate (HR) in 6-week swimming exercised compared with sedentary mice. (b) Consistent with increased parasympathetic nerve activity (PNA), 6-week swimming exercised mice had increased high frequency (HF) power compared with sedentary mice. The relation between heart rate and HF power is shown.R2=0.63 sedentary and 0.49 for exercised, Pearson’sP<0.01 in both groups. (c) The change in atrial effective refractory period (AERP) after atropine was greater in exercised mice compared with sedentary. (d) Atropine reduced the duration of AF in exercised mice, suggesting a role of PNA in AF susceptibility in exercised mice. Treadmill exercised mice are shown by circles and swimming exercised mice by squares. Thenvalues indicate number of mice used. Data presented as mean±s.e.m.*P<0.05 compared with sedentary using unpaired Student’st-test. **P<0.05 compared with sedentary using paired Student’st-test.#P<0.05 using one-way ANOVA. Figure 3: Effects of atropine on AF susceptibility in exercised mice. ( a ) Administration of 2 mg kg −1 atropine had a larger effect on heart rate (HR) in 6-week swimming exercised compared with sedentary mice. ( b ) Consistent with increased parasympathetic nerve activity (PNA), 6-week swimming exercised mice had increased high frequency (HF) power compared with sedentary mice. The relation between heart rate and HF power is shown. R 2 =0.63 sedentary and 0.49 for exercised, Pearson’s P <0.01 in both groups. ( c ) The change in atrial effective refractory period (AERP) after atropine was greater in exercised mice compared with sedentary. ( d ) Atropine reduced the duration of AF in exercised mice, suggesting a role of PNA in AF susceptibility in exercised mice. Treadmill exercised mice are shown by circles and swimming exercised mice by squares. The n values indicate number of mice used. Data presented as mean±s.e.m. * P <0.05 compared with sedentary using unpaired Student’s t -test. ** P <0.05 compared with sedentary using paired Student’s t -test. # P <0.05 using one-way ANOVA. Full size image Figure 4: Increased action potential durations and I Ca in the atria of exercised mice. ( a ) Representative averaged action potentials recorded using sharp microelectrode in isolated ex vivo atria from sedentary and swimming exercised mice. ( b ) Six weeks of exercise increased the average time to 30, 50 and 90% repolarization (APD30, APD50 and APD90) of left atrial myocytes. N =21/6 mice for sedentary, n =23/6 mice for exercise. ( c ) Representative I Ca recordings in left atrial myocytes using whole-cell patch-clamp. ( d ) I Ca I-V curves in left atrial myocytes showing increase in I Ca in 6-week exercised mice; n =14 myocytes/3 mice for exercised and n =12/3 mice for sedentary. ( e ) Increased RyR2 phosphorylation at S2814 in atria of 6 week (6w) and four session (4x) swim exercised mice as compared with sedentary (Sed) mice. Please note the reduction in RyR2 phosphorylation in the ventricles of 6-week swim exercised mice. The n values indicated on bar graph and represent number of mice. ( f ) Ca 2+ spark activity in the atria of swim and sedentary exercised mice with representative spark activity shown in top panel; n =35/3 mice for sedentary, n =42/3 mice for exercise. Scale bar, 200 ms. Data presented as mean±s.e.m. * P <0.05 compared with sedentary at the same membrane potential using Student’s t -test. ** P <0.01 compared with sedentary using Student’s t -test. # P <0.05 using one-way ANOVA. Full size image Structural remodelling in atria of exercised mice The inability of PNA blockade to entirely prevent AF vulnerability in exercised mice combined with the increased AF incidence in isolated denervated exercised atria motivated us to examine other factors previously linked to AF including atrial enlargement [8] , interstitial collagen deposition (fibrosis) [32] and inflammation [10] , [33] . Exercised mice increased ( P =0.01, Student’s t -test) interstitial collagen deposition ( Fig. 5a,b ) in atria without differences ( P =0.4, Student’s t -test) in ventricles. As tissue fibrosis is invariably associated with inflammation in AF [10] , [33] , cardiac sections were examined with toluidine blue (Mast cells), Ly6b.2 antibodies (primarily neutrophils and recently activated inflammatory monocytes [34] ) and Mac-3 antibodies (macrophages and monocytes). Although no elevations in mast cells or Ly6b.2-positive cells were observed acutely (2 days) or after 6 weeks of exercise training, Mac-3-positive macrophage/monocyte numbers were increased ( P =0.005, Student’s t -test) after 6 weeks of exercise ( Fig. 5c,d ). Increased macrophage/monocyte numbers, without neutrophil infiltration, support the conclusion that inflammation in exercised atria does not result from inflammatory cell infiltration as might occur with myocyte damage. No differences ( P =0.67, Student’s t -test) in staining patterns (Ly6b.2 and Mac-3 staining) were observed in ventricles between exercise (16.26±2 cells mm −2 ) and sedentary mice (14.1±4 cells mm −2 ). We also observed increased ( P =0.03, n =3, Student’s t -test) fibroblast numbers in atria from mice after 6 week of swimming (887±135 cells mm −2 ) compared with sedentary controls (409±55 cells mm −2 ), without evidence of myofibroblasts positive for α-smooth muscle actin staining. In addition to fibrosis and inflammation, we observed atrial hypertrophy ( P =0.02, Student’s t -test), measured as atrial-to-ventricular weights or atria-to-body weights ratios, in mice after 6 weeks of swimming ( Table 1 ). There was no change in absolute left ventricle weights or left ventricle weights normalized to tibia length ( Table 1 ), but we did observe a slight increase in left ventricle weights normalized to body weights ( Table 1 ) as previously shown in exercised mice [35] . Consistent with atrial hypertrophy, whole-cell patch-clamp measurements also revealed increased ( P =0.01, Student’s t -test) atrial capacitance in the swimming (74.4±2.4 pF, n =46) compared with sedentary groups (66.2±2.3 pF, n =48). 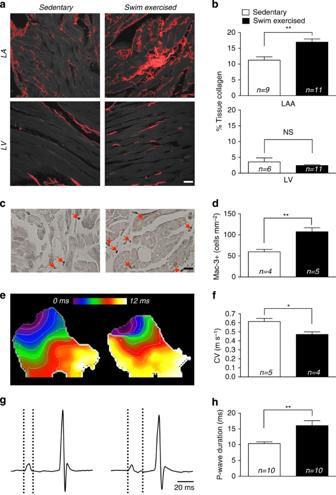Figure 5: Increased interstitial fibrosis and inflammation in atria of swimming exercised mice. (a) Representative images of picrosirius red-stained hearts showing increased myocardial collagen in atria but not ventricles of exercised mice (red). (b) Summary of % tissue collagen derived from picrosirius red stained sections. (c) Representative Mac-3-stained atrial sections showing increased macrophage counts with exercise (shown by red arrows). (d) Normalized macrophage counts. (e) Isochronal activation maps of paced left atrial appendages showing time to activation of the left atrial appendage from site of stimulation. (f) Averaged conduction velocities (CV) calculated from activation maps of the left atrial appendage. (g) Representative surface ECG recordings showing prolonged P-wave durations in exercised mice (dashed line). In all, 55% of exercised compared with 10% of sedentary mice showed +/− p-wave morphology. (h) Average P-wave durations. Thenvalues indicated on bars represent number of mice used. Data presented as mean±s.e.m. *P<0.05 when exercised is compared with sedentary using Student’st-test. **P<0.05 when exercised is compared with sedentary using Welch’st-test. Scale bars indicate 100 μm. NS, not significant. Figure 5: Increased interstitial fibrosis and inflammation in atria of swimming exercised mice. ( a ) Representative images of picrosirius red-stained hearts showing increased myocardial collagen in atria but not ventricles of exercised mice (red). ( b ) Summary of % tissue collagen derived from picrosirius red stained sections. ( c ) Representative Mac-3-stained atrial sections showing increased macrophage counts with exercise (shown by red arrows). ( d ) Normalized macrophage counts. ( e ) Isochronal activation maps of paced left atrial appendages showing time to activation of the left atrial appendage from site of stimulation. ( f ) Averaged conduction velocities (CV) calculated from activation maps of the left atrial appendage. ( g ) Representative surface ECG recordings showing prolonged P-wave durations in exercised mice (dashed line). In all, 55% of exercised compared with 10% of sedentary mice showed +/− p-wave morphology. ( h ) Average P-wave durations. The n values indicated on bars represent number of mice used. Data presented as mean±s.e.m. * P <0.05 when exercised is compared with sedentary using Student’s t -test. ** P <0.05 when exercised is compared with sedentary using Welch’s t -test. Scale bars indicate 100 μm. NS, not significant. Full size image These structural changes in atria from exercised mice were associated with slowed ( P =0.02, Student’s t -test) conduction velocities and prolonged ( P =0.003, Student’s t -test) P-wave durations ( Fig. 5e–h ) without changes in either connexin-40 or connexin-43 expression in swimming mice compared with sedentary mice ( Supplementary Fig. 12 ). Interestingly, the organizational index of ECG recordings during AF episodes in exercised atria were greater, consistent with models of structural remodelling in AF [22] ( Supplementary Fig. 7 ). Importantly, if we examined mice 6 weeks after the termination of the 6-week swim training, the atrial AF vulnerability and fibrosis persisted ( P =0.02, Student’s t -test), while HR changes were reversed after detraining (to 492±7 beats/minute, P =0.02 compared with 6 weeks swim exercised, Student’s t -test), establishing that the exercise-induced structural remodelling is not readily reversible ( Supplementary Fig. 13 ). Role of TNFα in exercise-induced atrial structural remodelling To gain insight into the possible genetic and biochemical mechanisms underlying exercise-induced AF, we performed gene set enrichment analysis (GSEA) of microarray gene expression values that revealed enrichment of several signalling pathways (p38 MAPK and NFκB pathways) associated with inflammation in exercised atria ( Supplementary Fig. 14A,B , Supplementary Table 5 ). Although these enriched pathways are regulated by several factors [36] , [37] , they are nevertheless downstream of, or cross-talk with, TNFα [36] , [38] . These observations, combined with previous studies implicating TNFα in the promotion of AF [19] , [39] , suggest that TNFα plays a role in AF pathogenesis with exercise. In support of this possibility, acute bouts of exercise activated ( P =0.03, Student’s t -test) NFκB, the canonical downstream transcription factor of TNFα, in atria, but not in ventricles ( P =0.2, Fig. 6a,b , Student’s t -test). Acute bouts of exercise also increased the phosphorylation levels of other downstream factors of TNFα signalling such as IκB ( P =0.01, Student’s t -test) and p38 MAPK ( P =0.03, Student’s t -test) compared with sedentary controls ( Fig. 6c,d ). 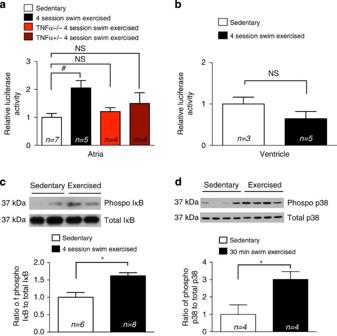Figure 6: Increased NFκB binding activity and p38 phosphorylation with swimming exercise. (a) NFκB-driven luciferase activity was measured in atria and ventricles after four sessions of swimming exercise in wildtype,TNFα+/−andTNFα−/−mice (see methods). Values were normalized to protein concentration. (b) No change in NFκB luciferase activity was observed in the ventricle of exercised mice. (c) IκB phosphorylation increased 2 h post swimming exercise. Mice were exercised for four sessions, and atria were isolated 2 h after final exercise session. Summary bar graphs showing phosphorylated IκB normalized to total endogenous IκB. (d) P38 phosphorylation increased following 30 min of swimming exercise. Mice were exercised for 30 min and the atria were rapidly isolated and probed for p38 phosphorylation using western blots. Summary data of phosphorylated p38 normalized to total p38 are shown. Thenvalue shown on bar graphs and present number of mice used. Data presented as mean±s.e.m. *P<0.05 using student’st-test.#P<0.05 using one-way ANOVA. NS, not significant. Figure 6: Increased NFκB binding activity and p38 phosphorylation with swimming exercise. ( a ) NFκB-driven luciferase activity was measured in atria and ventricles after four sessions of swimming exercise in wildtype, TNF α +/− and TNF α −/− mice (see methods). Values were normalized to protein concentration. ( b ) No change in NFκB luciferase activity was observed in the ventricle of exercised mice. ( c ) IκB phosphorylation increased 2 h post swimming exercise. Mice were exercised for four sessions, and atria were isolated 2 h after final exercise session. Summary bar graphs showing phosphorylated IκB normalized to total endogenous IκB. ( d ) P38 phosphorylation increased following 30 min of swimming exercise. Mice were exercised for 30 min and the atria were rapidly isolated and probed for p38 phosphorylation using western blots. Summary data of phosphorylated p38 normalized to total p38 are shown. The n value shown on bar graphs and present number of mice used. Data presented as mean±s.e.m. * P <0.05 using student’s t -test. # P <0.05 using one-way ANOVA. NS, not significant. Full size image To more directly assess the involvement of TNFα in exercise-mediated atrial remodelling, the pharmacological inhibitor of TNFα etanercept (Enbrel) and mice lacking the TNFα gene ( TNF α −/− ) were studied. Interference with TNFα abolished the exercise-induced increases in NFκB-driven luciferase activity ( Fig. 6a ), the increased susceptibility to AF ( Fig. 7a,c , Supplementary Fig. 5D ), atrial fibrosis ( Fig. 7b,d ) and increases in Mac-3-positive cells ( Fig. 8 ). Interestingly, when etanercept treatment was started 3 weeks post swimming exercise, neither atrial fibrosis nor AF susceptibility was prevented ( Supplementary Fig. 13C,D ). 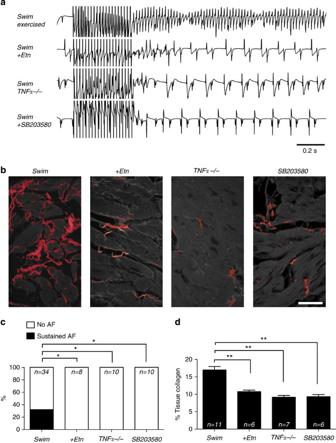Figure 7: TNFα and p38 inhibition prevents arrhythmogenic atrial remodelling. (a) Representative atrial arrhythmia induction in untreated, etanercept (Etn) treated,TNFα knockout (−/−) and p38 inhibitor SB203580 treated mice swimming exercised for 6 weeks. (b) Representative picrosirius red-stained atrial sections showing prevention of fibrosis (red) in exercised etanercept treated, exercisedTNFα−/−and exercised SB203580 treated mice compared with untreated exercised mice. (c) Percentage of mice showing sustained AF episodes. Sustained episodes of AF were not induced in etanercepttreated,TNFα−/−or SB203580-treated mice with exercise. (d) Summary data showing percent fibrosis in exercised etanercept treated, exercisedTNFα−/−and SB203580 treated mice. Thenvalue shown on bar graphs and present number of mice used. Data presented as mean±s.e.m.χ2-test *P<0.05 when exercised untreated is compared with exercised+Etn, exercisedTNFα−/−or exercised SB203580 treated mice. **P<0.05 when exercised untreated is compared with exercised+Etn, exercisedTNFα−/−, or exercised SB203580 treated mice using one-way ANOVA with Dunnett’smultiple comparison test. Scale bar, 100 μm. Interference with TNFα ( TNF α −/− ) also prevented the increased atria-ventricular weight ratios ( Supplementary Table 6 ) without affecting either the mild ventricular chamber dilation or HR reductions induced by exercise ( Supplementary Table 7 ). Moreover, APD prolongation ( P <0.01, Student’s t -test) was also seen with exercise in TNF α −/− atrial myocytes, with no change in the amplitude or resting membrane potentials ( Supplementary Fig. 10E–H ). Figure 7: TNFα and p38 inhibition prevents arrhythmogenic atrial remodelling. ( a ) Representative atrial arrhythmia induction in untreated, etanercept (Etn) treated, TNF α knockout ( −/− ) and p38 inhibitor SB203580 treated mice swimming exercised for 6 weeks. ( b ) Representative picrosirius red-stained atrial sections showing prevention of fibrosis (red) in exercised etanercept treated, exercised TNF α −/− and exercised SB203580 treated mice compared with untreated exercised mice. ( c ) Percentage of mice showing sustained AF episodes. Sustained episodes of AF were not induced in etanercepttreated,TNFα −/− or SB203580-treated mice with exercise. ( d ) Summary data showing percent fibrosis in exercised etanercept treated, exercised TNF α −/− and SB203580 treated mice. The n value shown on bar graphs and present number of mice used. Data presented as mean±s.e.m. χ 2 -test * P <0.05 when exercised untreated is compared with exercised+Etn, exercised TNF α −/− or exercised SB203580 treated mice. ** P <0.05 when exercised untreated is compared with exercised+Etn, exercised TNF α −/− , or exercised SB203580 treated mice using one-way ANOVA with Dunnett’smultiple comparison test. Scale bar, 100 μm. 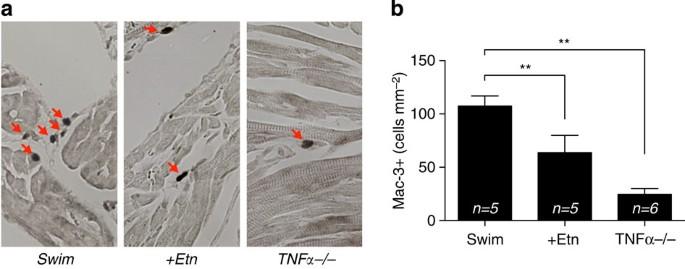Figure 8: Reduced inflammation with TNF inhibition. (a) Representative Mac-3-stained atrial sections for macrophages/monocytes (shown by red arrows) showing prevention of macrophage/monocyte count increases in exercised etanercept treated and exercisedTNFα−/−mice compared with untreated exercised mice summarized in (b). Thenvalue shown on bar graphs and present number of mice used. Data presented as mean±s.e.m. **P<0.05 when exercised untreated is compared with exercised+Etn or exercisedTNFα−/−using one-way ANOVA with Dunnett’smultiple comparison test. Scale bar, 100 μm. Full size image Figure 8: Reduced inflammation with TNF inhibition. ( a ) Representative Mac-3-stained atrial sections for macrophages/monocytes (shown by red arrows) showing prevention of macrophage/monocyte count increases in exercised etanercept treated and exercised TNF α −/− mice compared with untreated exercised mice summarized in ( b ). The n value shown on bar graphs and present number of mice used. Data presented as mean±s.e.m. ** P <0.05 when exercised untreated is compared with exercised+Etn or exercised TNF α −/− using one-way ANOVA with Dunnett’smultiple comparison test. Scale bar, 100 μm. Full size image Previous studies have shown that increased fibrosis is linked to TNFα and p38 activation [40] , and we found that p38 phosphorylation was acutely elevated by exercise ( Fig. 6d ) in addition to the observed chronic differential expression of p38 pathway related genes ( Supplementary Table 5 ). Consistent with a role for p38 activation in exercise-induced remodelling, treatment of mice with the p38 inhibitor SB203580 during the 6-week exercise period completely prevented AF ( P =0.021, Fig. 7a,c , χ 2 -test) as well as atrial fibrosis ( P <0.01, Fig. 7b,d , one-way ANOVA). In addition, the acute exercise-induced elevation in p38 phosphorylation was significantly reduced in TNF α −/− mice ( P =0.5, Supplementary Fig. 14C , Student’s t -test) supporting the conclusion that exercise induces atrial-selective remodelling via TNFα-dependent p38 activation. Our results support the conclusion that increased PNA and structural atrial remodelling, characterized by inflammation, hypertrophy and fibrosis, increase AF vulnerability in intense exercised mice. Our studies show that the mechanosensitive inflammatory cytokine TNFα is central to the pathophysiology of AF induced by intense exercise but does not appear to interfere with the beneficial physiological ventricular remodelling as well as the electrical remodelling seen with exercise. Involvement of TNFα in exercise-induced atrial remodelling is supported by the enrichment of the p38 and NFκB pathways [36] , [37] , [38] in our microarray analysis, by increased IκB and p38 phosphorylation in atrial lysates, and by elevated NFκB activity in atria, but not ventricles, following acute bouts of exercise. Although altered TNFα-dependent signalling can occur with or without changes in TNFα levels, or TNFα shedding [41] , we were unable to determine whether atrial TNFα levels change with exercise because the specificity of commercially available antibodies could not be verified by us (using TNF α −/− heart lysates). Although our studies focused primarily on swimming-based exercise in mice, we also observed similar responses to exercise in mice undergoing tread-mill running (that is, reduced heart rates, mild ventricular hypertrophy, increased vagal tone, increased incidence of AF both in vivo and ex vivo , and increased fibrosis in atria but not ventricles). Although we did not fully explore the role of TNFα in the response of mice to tread-mill running, the similar responses in the swimming and tread-mill running mice suggested that interference with TNFα will also be effective in treadmill exercised mice that will require further studies to validate. Involvement of TNFα-dependent pathways readily explains the structural atrial remodelling with exercise since TNFα is an integral component of inflammatory responses, by recruiting circulating monocytes [42] and regulating resident tissue macrophages [43] . In addition, TNFα is a central regulator of cardiac hypertrophy [19] and fibrosis that involves altered p38 activity in fibroblasts [17] , [44] . In this regard, we found that pharmacological blockade of p38, as with TNFα inhibition, also prevented AF and structural remodelling without interfering with the physiological changes in heart rate and the ventricular chambers induced by exercise. The underlying mechanisms for the activation of these pathways and the differential pathological remodelling on atria versus ventricles with exercise are unclear. However, stretch has been shown to activate TNFα in cardiac [17] , [18] , skeletal [45] , fibroblasts [46] and smooth muscle [47] cells, and we noted that exercise in mice leads to sharp elevations in diastolic atrial pressures exceeding 30mmHg ( Supplementary. Fig. 15 ), as seen in humans [15] . Although the pericardium constrains heart volumes, the atrium expansion is (~2-fold) greater than ventricular expansion under conditions when the pericardium becomes engaged [48] , and this may underlie the rise in serum TNFα [14] as well as serum atrial natriuretic peptide [49] seen in exercising humans. A role for stretch in atrial remodelling resulting from intense exercise in our mice is supported by our findings that atria have a far greater compliance than ventricles ( Supplementary Fig. 15 ) as well as by previous studies showing that atrial fibroblasts undergo transformation to proliferating, collagen-secreting myofibroblasts in response to stretch more easily than ventricular fibroblasts [50] . However, exercise induces a multitude of metabolic, biochemical and physiological changes in multiple cells types that could lead to stretch-independent activation of TNFα and its downstream signalling molecules like p38 (ref. 51 ). Clearly, additional studies will be required to address the underlying mechanisms for TNFα/p38-mediated atrial remodelling with exercise. In this regard, we are currently examining the effects of tissue-specific TNFα deletion including immune cell deletions on exercised-induced atrial remodelling in our mice. Our findings predict that interference with, or reductions in, TNFα-dependent signalling pathways could prove useful in minimizing the harmful consequences of intense exercise on atria, without interfering with either the performance of endurance athletes or the many otherwise highly beneficial effects of exercise. Nevertheless, since previous clinical trials with etanercept in advanced heart failure patients were terminated due to a lack of efficacy [52] , despite showing promise in animal studies [53] , etanercept may have limited efficacy in preventing detrimental atrial remodelling with exercise, even though etanercept is equally effective in animals and human in other diseases, such as rheumatoid arthritis [54] . It is worth noting that, although treating mice with human-based etanercept is expected to evoke an immune response, intraperitoneal injection of etanercept has been used often in animal models to treat TNFα-dependent inflammatory conditions [53] , [54] . The modulation of pathways downstream of TNFα such as p38 might also represent viable targets for future interventions. In this regard, p38 inhibitors have been used in heart failure models and shown to reduce cardiac apoptosis and fibrosis in the ventricles [55] . These findings are intriguing because acute bouts of exercise elevated p38 phosphorylation, and chronic p38 inhibition prevented the adverse structural remodelling in the atria associated with 6 weeks of exercise. It should be mentioned that inhibition of the PNA reduced, but did not eliminate AF susceptibility in exercised mice. PNA involvement in exercise-induced AF is anticipated based on its link to AF in endurance athletes [56] , which presumably occurs via effects on atrial ERP (via I K,Ach ). Consistent with this possible mechanism, our exercised mice had signs of elevated PNA (that is, elevated heart rate variability and lower heart rates), similar to that seen in human athletes [11] . Indeed, following PNA blockade, atrial ERPs prolonged more in exercised mice compared with controls and these differences correlated with longer APDs in cardiomyocytes from exercised mice that were not associated with alterations in K + currents but were linked to enhanced L-type Ca 2+ currents (I Ca,L ), as was also reported previously in ventricular myocytes due to changes in PI3Kinase signalling with exercise [57] . Our studies also uncovered modest increases in RyR2 phosphorylation at position S2814 (but not S2808) following swimming exercise that was accompanied by trends towards increased spontaneous Ca 2+ spark activity in atria. Increased RyR2 phosphorylation and Ca 2+ leak as a result of CaMKII activation has previously been reported in human AF patients [26] , [27] as well as mouse AF models [28] . In this regard, CaMKII can be activated by a number of inflammatory factors, including TNFα [58] , as well as a number of inter-related mechanisms including elevated Ca 2+ and oxidative stress [59] . Interestingly, we did not observe any changes in CaMKII phosphorylation at T287 or expression levels of CaMKII with exercise, although recent studies have questioned the specificity of CaMKII phospho-specific antibodies [60] . Future studies will clearly be required to determine the roles and links between RyR2, CaMKII and TNFα in atrial remodelling induced by exercise. As seen in our exercised mice, human athletes also show reductions in heart rate mediated by changes in autonomic nerve activity that reverse after long-term deconditioning [61] , while chamber dilatation persists. In contrast, it remains unknown whether cessation of exercise can eliminate the atrial remodelling and AF vulnerability. In this regard, we found that reversal of atrial fibrosis and enhanced vulnerability to atrial arrhythmias persisted after 6 weeks after cessation of swimming exercise (for 6 weeks), despite the reversal of HR slowing as in human. If these observations are applicable to humans, they highlight the critical importance of identifying and interfering with pro-fibrotic pathways activated by exercise. These results further suggest that exercise as well as other factors inciting atrial structural remodelling (such as hypertension, valve disease, heart failure) may accumulate with age, which readily explains the strong link between age and AF [62] including in endurance athletes [63] . On the other hand, it is clearly conceivable that ageing could influence the response of the atria to stresses induced by exercise and other cardiovascular conditions. Nevertheless, consistent with the potentially cumulative and irreversible nature of atrial structural remodelling, we failed to prevent the increased fibrosis in the atria of exercised mice when treatment with etanercept was started (3 weeks after initiating swimming exercise). Interestingly, many studies have established that ageing and cardiovascular disease are themselves accompanied by inflammation, with TNFα being involved in both conditions [64] . Future studies that are designed to identify individuals at risk for exercise-induced AF should develop methodologies for the longitudinal assessment of atrial remodelling in athletes. It is also imperative for future studies to identify the training and exercise conditions (intensity, duration, frequency) that most strongly predispose to pathological atrial remodelling; we are currently engaged in studies designed to address precisely these questions in our mouse models. Despite the similar AF and fibrosis between our results and exercised rats [7] , the extrapolation of rodent results to human athletes clearly requires caution. Besides having much smaller hearts, mice also have 10-fold greater HRs than humans, thus potentially making mice less susceptible to arrhythmias. Nevertheless, the ERPs in mice are also proportionally shorter, which probably explains the many previous mouse studies that reproduce human cardiac arrhythmias. Another notable difference between humans and mice, of particular relevance to our studies, is the relative differences in heart rate increases during exercise; in humans, heart rate can be increased by 3–4 times above baseline heart rates while in mice the heart rates increase by only ~50%. Consequently, mice are expected to rely much more on stroke volume increases in order to elevate cardiac output during exercise compared with humans. If atrial stretch is indeed a major factor in atrial remodelling, then exercise is predicted to create a far stronger stimulus for atrial remodelling in mice compared with humans. While these species differences in response to exercise could explain the appearance of atrial hypertrophy and inflammation after only 6 weeks of intense exercise, it is also important to note that the atrial filling pressures changes during exercise are remarkably similar in mice and humans (that is, compare Supplementary Fig. 15A with Reeves et al . [15] ). It should be mentioned that our exercise programmes were not voluntary. Nevertheless, stress was minimized in our exercised mice in several ways. Mice swam against a water current thereby avoiding the drowning stress associated with tail-weights, bubbling or mild detergents to break the surface tension of water. In addition, with the treadmill exercise, the use of electrical shocks was limited to the pre-training sessions and not used during the remainder of the exercise protocol. We believe that stress is not a major factor in the atrial remodelling in the mice for several reasons. First, the HR in our animals decline as early as 1 week after the start of the exercise protocol, whereas mice subjected to psychosocial stress show chronic HR elevations [65] . Second, though fecal corticosterone levels tended to be higher in exercised versus sedentary mice, the difference was not significant ( Supplementary Fig. 1B ). The interpretation of these corticosterone measurements is complicated because acute and chronic [66] intense exercise in humans independently causes elevated cortisol levels. Additional studies are needed to understand the link between stress, exercise and AF induction. Experimental animals and exercise protocols All mice were housed at the Division of Comparative Medicine animal facility in accordance with the standards of the Canadian Council on Animal Care. Ethical approval for all animal experiments was granted by the University of Toronto. In preliminary studies we found that CD1 strain of mice (Charles River Laboratories) instinctively swim against a current in our swimming apparatus, a behaviour that was found to be absent in other strains. In studies using mice with whole-body TNFα disruption (c57b, Taconic model #1921) or expressing an NFκB-Luc reporter (c57b, Jackson Laboratories stock #006100), a single back-cross with CD1 mice was sufficient to manifest instinctive swimming behaviour. Mice swam in water containers (30 cm diameter) with a steady water current (325 l min −1 ) generated by a central water pump at 34 °C. Swimming training began with 30-min swimming sessions (twice daily, separated by 4 h) that were increased to 90 min by adding 10 min per day. Training then continued for 6 weeks. For running exercise, mice trained on a treadmill apparatus (Harvard Apparatus) at 35 cm s −1 with a 30° incline. Running training began with 30-min sessions (once daily) that were increased by 10 min per day to 120 min. In the first 3–4 sessions, electric stimulation (0.2 mA) was used to promote running during training; thereafter, mice were encouraged to run using a soft brush pressed against their posterior region, to reduce the potential stress of continued electric shocking. Male mice were randomly assigned to exercised or sedentary groups at 6 weeks of age. No mice were excluded from the study based on inability to train. Control animals were placed in water containers without water current for 5 min, or placed on the treadmill for 5 min at 5 cm s −1 . Mice treated with etanercept (Enbrel) were injected subcutaneously daily at 2.5 mg kg −1 for the entire 6-week exercise training. Mice treated with SB203580 (AbMole Bioscience) were injected i.p. at 4 mg kg −1 . All experimental assessments were conducted 24 h after the final exercise session. The identity of the groups (exercised versus sedentary) was concealed to the investigators. Sample sizes were determined using power calculations at 95% confidence interval and 80% power using comparable data from previously published results [67] . VO 2 consumption measurements Oxygen consumption was determined using Oxymax oxygen monitoring (Columbus instruments, Columbus, OH). For swimming, mice were placed in a sealed container containing water pumps to generate current (34 °C). Maximal O 2 consumption was determined using the swimming apparatus with two simultaneous pumps generating current on opposite ends. We have found that mice in this set-up consume the greatest amount of O 2 (11260±563 ml kg −1 h −1 ), which was much greater than values that could be obtained using exhaustive treadmill exercise with speeds of up to 50 cm s −1 and 30° incline (9384±643 ml kg −1 h −1 ). Echocardiography Mice were anaesthetized using 1.5% isoflurane oxygen mixture. Mice were placed on a heating pad and body temperature was maintained between 36.9 and 37.3 °C for the duration of the measurements. Transthoracic M-mode echocardiographic examination was conducted using a Vevo 7700 system (VisualSonics) equipped with ultrasonic linear transducer scanning heads operating at 30 MHz. The left ventricular long axis view was used for measurement of chamber size and wall diameter. Data analysis was performed using the VisualSonics data analysis suite. Electrocardiography Surface ECG measurements were conducted on mice anaesthetized using a 1.5% isoflurane oxygen mixture with sub-dermal platinum electrodes placed in lead II arrangement. Body temperature was maintained at 36.9 to 37.3 °C. To record heart rates from unanaesthetized, unrestrained animals, radiofrequency emitting ECG units (Data Sciences International) were implanted in the intraperitoneal cavity and the electrodes placed in lead II arrangement subdermally. After 1 week of recovery, mice were exercised according to the standard regimen and heart rate (HR) was recorded weekly over a 48-h period. Data were analysed using Ponemah Physiology Platform software. To assess pharmacological inhibition of autonomic nerve activity, HRs of anaesthetized mice were monitored before and after intraperitoneal injection of 2 mg kg −1 BW of atropine sulphate and 10 mg kg −1 BW of propranolol hydrochloride (Sigma-Aldrich) to block the parasympathetic and sympathetic branches of the autonomic nervous system. Heart-rate variability analysis Minimum anaesthesia deepness was strictly monitored and maintained at equivalent levels between sedentary and exercised mice using the toe pinch-pedal reflex. Surface ECG recordings were marked for R-R intervals using P3 Plus (Data Sciences International), and the raw text files of the inter-beat-intervals (IBI) were input for analysis using Kubios HRV software (University of Eastern Finland). Frequency bands of 0–0.1 Hz and 0.1–5 Hz for low and high frequency components, respectively, were determined in a series of preliminary experiments ( Supplementary Fig. 9 ) using atropine (2 mg kg −1 ) and propranolol (10 mg kg −1 ). An interpolation rate of 20 Hz, with 256 point window was used to generate frequency domain plots. The absolute power from the frequency domain plot was used for analysis. A minimum of 5 min of data were used for the analysis. Assessment of electrical properties and arrhythmia vulnerability of hearts Mice were anaesthetized using 1.5% isoflurane and oxygen mixture, and a 2.0 French octapolar recording/stimulation electrophysiology catheter (CI’BER Mouse, Numed) was inserted into the right jugular vein and advanced into the right ventricle. The his bundle signal was used for consistent positioning of the catheter (see Supplementary Fig. 4 ). Appropriate leads were used to deliver programmed stimulation to either the right atria or right ventricle. All stimulations were delivered at a voltage magnitude of 1.5 times capture threshold, with 1 ms pulse duration. Refractory periods were determined by delivering seven pulses at 20 ms below the R-R interval followed by extrastimulation. The S2 coupling interval was initially delivered at below capture (~15 ms) and increased by 5 ms increments until capture. The coupling interval was reduced by 1–2 ms again until loss of capture. Our protocols for arrhythmia were based on previously published protocols using burst pacing with intervals less than atrial effective refractory in both exercise and sedentary mice ( Supplementary Table 4 ). For arrhythmia induction, 27 pulses (of 2 ms duration) at 40 ms intervals were applied to the right atrium or ventricle and reduced to 20 ms intervals by 2 ms decrements, repeated three times. If arrhythmia events were not induced, 20 trains (applied every 1.5 s) of 20 pulses (2 ms duration) with an interpulse interval of 20 ms duration were used. Sustained arrhythmias were defined as reproducible episodes of rapid, chaotic and continuous atrial or ventricular activity, lasting longer than 10 s (examples in Supplementary Fig. 6 ). Optical mapping and intracellular action potential recording Heparinized mice were anaesthetized using isoflurane and killed via cervical dislocation. The thorax was opened by midsternal incision, and the heart was excised into warm (35 °C) Tyrode’s solution (in mmol/l): 140 NaCl, 5.4 KCl, 1.2 KH 2 PO 4 , 1 MgCl 2 , 1.8 CaCl 2 , 5.55 D -glucose, 5 HEPES and 10 U ml −1 heparin (pH 7.4). The heart was pinned to a Sylgard coated petri dish with insect pins to reveal the dorsal atrioventricular connective tissue. The pericardium and any other residual lung and connective tissue were carefully excised from the heart. A small lining of adipose tissue guided incisions along the atrioventricular connective tissue until complete separation of the atria from the ventricles was achieved. Atria were then pinned so as to reveal the mitral and tricuspid valves. Fine scissors were inserted into the superior and inferior vena cava, and incisions were made in a straight path to ‘open’ the atria. The atria were then turned to reveal the pulmonary veins, and residual lung tissue was removed. Atria were then transferred and continuously superfused using 35 °C carbogenized (95% O 2 & 5% CO 2 ) Krebs solution (in mmol l −1 ): 118 NaCl, 4.2 KCl, 1.2 KH 2 PO 4 , 1.5 CaCl 2 , 1.2 MgSO 4 , 2.3 NaHCO 3 , 20 D -glucose, 2 Na-pyruvate (pH measured at 7.35–7.4). For optical mapping measurements, isolated atrial preparations were stained with 10 μM voltage-sensitive dye Di-4-ANEPPS (Sigma-Aldrich) for 10 min and then superfused continuously with carbogenized Krebs solution (35 °C). The flow rate, volume and temperature of the solution was kept constant throughout and in-between the experiments. The pH of the bath solution in the perfusion vessels was monitored to ensure that the pH was between 7.35 and 7.4. To calculate conduction velocity, atria were paced at 90 ms interval from the left atrial appendage, and images were captured at 1408 frames s −1 using a high speed camera (Photometrics, AZ, USA). Activation maps were generated to calculate conduction velocity. To induce atrial arrhythmias, the same stimulation protocols that were used in vivo using intracardiac catheter were applied. Sustained arrhythmias were defined as a reproducible episode of rapid, chaotic atrial activation lasting longer than 10 s. Images were acquired using ImagePro Plus software (Mediacy) and analysed using ImageJ or Scroll (custom software) [68] , which was modified to perform phase analyses. For intracellular action potential recordings, pipettes were pulled from borosilicate glass using a Flaming/Brown pipette puller (Sutter Instrument Company). Pipettes were filled with 3 M KCl solution and the resistance was between 30 and 50 MΩ. Intracellular recordings of atrial myocytes (in tissue, not isolated) were acquired by placing the microelectrodes into the left atrial appendage. ClampFit software (Axon) was used for analysis. Isolation of atrial myocytes and I Ca measurement Left atrial myocytes were obtained from 6-week exercised and age-matched sedentary (CD-1, male 14 weeks old) mice. Mice were anaesthetized with 2.5% isoflurane, and hearts were removed rapidly and retrograde perfused with Ca 2+ -free Tyrode’s solution (mM): 137 NaCl, 5.4 KCl, 1.0 MgCl 2 , 10 D -Glucose, 10 HEPES, pH 7.4 at 37 °C through the aorta for 10 min. After perfusing the heart with collagenase (1.0 mg ml −1 , Worthington) and elastase (0.2 mg ml −1 , Worthington) for 8–10 min, the left atrial appendage was dissected and stored in Kraftbruhe (KB) buffer (mM): 120 potassium glutamate, 20 KCl, 20 HEPES, 1.0 MgCl 2 , 10 D-glucose, 0.5 K-EGTA, 0.1% bovine serum albumin, pH 7.4. Single myocytes were obtained by gently triturating the left atrial appendage using a polished glass pipette with a 5 mm opening for 6–10 min. Single atrial myocytes were stored in KB buffer at 4 °C until use. For recording Ca 2+ currents (I Ca ), single left atrial myocytes were superfused with bath solution containing (mM): 140 NaCl, 4 CsCl, 1 MgCl 2 , 1.5 CaCl 2 , 10 HEPES, 10 D -glucose (pH 7.3) for 10 min and only Ca 2+ tolerant cells were used for recording. I Ca was recorded using whole-cell patch clamp (Axopatch 200B and Clampex 8 software, Axon Instrument, CA, USA) at room temperature. The pipette resistance ranged between 4 and 6 MΩ when filled with internal solution, containing (in mM): 135 CsCl, 6 NaCl, 1 MgCl 2 , 3 MgATP, 10 HEPES and 10 EGTA (pH to 7.2 with CsOH). I Ca was recorded under voltage-clamp mode with 80% compensation of cell capacitance and series resistance. After membrane rupture, cell capacitance was measured by integrating capacitance transients initiated by 5 mV steps from holding potential of −50 mV and was used to normalize the magnitude of recorded currents. For recording I Ca , cells were held at −75 mV and stepped to −40 mV for 50 ms to inactivate voltage-gated Na + currents before stepping to test potentials from +50 mV to −40 mV decremented by 10 mV. For recordings acetylcholine-activated K + currents (I k,Ach ), single left atrial myocytes were superfused with bath solution containing (mM): 140 NaCl, 4 KCl, 1 MgCl 2 , 1.2 CaCl 2 , 10 HEPES, 10 D -glucose (pH 7.3) for 10 min and only Ca 2+ tolerant cells were used for recording. To block K ATP 10 μM Glybenclamide (Sigma) was added to the bath solution. Two different concentrations of carbachol (CCh, Sigma) were delivered to cells through 0.1 mm internal-diameter tubing sitting on top of the cells. The pipette resistance ranged between 4 and 6 MΩ when filled with internal solution, containing (in mM): 120 potassium aspartate, 20 KCl, 1 MgCl 2 , 3 MgATP, 0.1Na 2 GTP, 10 HEPES and 10 EGTA (pH 7.2). Cells were held at −70 mV and stepped to +30 mV for 120 s to ensure inactivation of all voltage-gated currents before addition of CCh for additional 120 s. I K,Ach current density was measured by subtracting baseline current before addition of CCh at +30 mV from maximal current induced by CCh addition normalized to cell size. Voltage-activated K + currents were recorded in bath buffer containing (mM): 140 NaCl, 4 KCl, 1 MgCl 2 , 1.2 CaCl 2 , 10 HEPES, 10 D-glucose and 0.3 CdCl 2 , pH 7.4. The pipette resistance ranged from 3 to 5 MΩ when filled with solution containing (mM): 120 K-aspartate, 20 KCl, 6 NaCl, 1 MgCl 2 , 3 MgATP, 10 HEPES, 10 EGTA, pH 7.4. Voltage-gated K + currents were measured by 20 s depolarization to +60 mV (close to reversal potential for sodium) from holding potential of −70 mV. Voltage-gated K + currents were analysed by fitting the decay phase of the outward K + currents to a three-exponential equation (equation (1)) to dissect the three components of outward K + current comprising of Ifast (I to ), intermediate (Kv1.5 encoded I K,slow1 ) and slow (Kv2-encoded I K,slow2 ). where A f , A i and A s are the amplitudes of the fast, intermediate and slow kinetic components decaying with time constants of τ f , τ i and τ s respectively. C is the amplitude of the steady-state, non-inactivating component. All data analysis was performed using ClampFit software (Axon). Histology Hearts were first perfused with saline containing 1% KCl followed by 4% paraformaldehyde in 0.1 M phosphate buffer. Hearts were embedded in paraffin and 5-μm thin sections were stained with Picrosirius red for visualization of collagen. Confocal laser scanning microscopy was used to image Picrosirius red stained sections (491 nm laser, 750 nm band pass emission), and imageJ software [69] was used for quantification. Perivascular and endocardial fibrosis were not included in the analysis for the quantification of % fibrosis. For quantitative measurement of macrophage infiltration, antibodies against mouse Mac-3 (1:200, BD Pharminogen, Cat. # 553322) were used with the streptavidin-biotin diaminobenzidine chromogen detection method (Vector Laboratories). Mac-3-positive cells were counted in three different sections (100 μm apart) of the left atrial appendage or left ventricle per replicate and standardized to the total tissue area of each slice. Images were acquired using Metamorph software (Molecular Devices), and data analysis was performed using ImageJ software. Mast cells were stained for using Toludine Blue at the appropriate PH. Mast cells were identified by metachromatic granules, counted and normalized to total tissue area. For quantitative measurement of connexin staining, heart sections were stained against connexin 40 (Abcam ab16585, 1:100 dilution) and 43 (Abcam ab11370, 1:100 dilution). Alexa Fluor 488 conjugated secondary antibody (Life technologies, 1:500 dilution) was used for connexin detection. Threshold method was used to determine number of pixels corresponding to connexin 40/43 staining and presented as value normalized to area of atria. Western blotting Atria and ventricles were isolated and frozen in liquid nitrogen. Protein was extracted in a cell lysis buffer consisting of 20 mM Tris-HCl, pH 7.5, 150 mM NaCl, 1 mM Na2EDTA, 1 mM EGTA, 1% Triton, 50 mM NaF, 1 mM Na3VO4, 1 mM PMSF, 2 mM Benzamindine, 1 μg ml −1 leupeptin. After centrifugation for 15 min at 12,000 × g , supernatants were extracted and protein concentration was determined using DCTM Protein Assay kit (1:1,000, #500–0112, BioRad, CA, USA). Forty micrograms of each sample was resolved by 12% sodium dodecyl sulphate–PAGE (SDS–PAGE) and transferred to nitrocellulose membranes. Blots were incubated with primary antibodies: phosphorylated p38 MAPK (1:1,000, PAB15917, Abnova, Taiwan, Supplementary Fig. 16A ), endogenous p38 MAPK (1:1,000, #9218, Cell Signaling Technology, USA, Supplementary Fig. 16B ), phosphorylated IκBα (1:2,000, 2859, Cell Signaling Technology, Supplementary Fig. 16C ), endogenous IκBα (1:1,000, #4814, Cell Signaling Technology, USA, Supplementary Fig. 16D ), and with secondary antibodies anti-rabbit (1:3,000, #7074, Cell Signaling Technology, USA) or anti-mouse (1:3,000, #7076, Cell Signaling Technology, USA). Phosphorylation of RyR2 was detected by using specific anti-S2814 RyR2 (1:1,000, Supplementary Fig. 16E ), S2808 RyR2 antibody (1:1,000, both in-house generated antibodies) and RyR2 antibody (1:1,000, Thermo scientific, Supplementary Fig. 16F ). Phosphorylation of CaMKII was detected by using a specific anti-pT286/287 CaMKII antibody (1:1,000, Cayman Chemical) and anti-CaMKII antibody (Epitomics). GAPDH was detected using an Anti-GAPDH antibody (1:1,0000, Millipore). Oxidation level of RyR2 was measured by oxyblot (OxyBlotTM Protein Oxidation Detection Kit, Millipore). Amersham ECL Prime Western Blotting Detection Reagent (RPN2232, GE Healthcare, UK) was used for detection, and analysis of bands was performed using densitometry plugin for ImageJ software. Ca 2+ spark activity Isolated left atrial myocytes were loaded with 1 μM fluo-3 Am at room temperature for 15 min followed by 15 min of desertification by continuously superfusing the cells with Tyrod’s buffer containing 1.2 mM Ca 2+ . After 15 min of desertification at room temperature, Ca 2+ tolerant cells were field stimulated at 1 Hz for 30 s at room temperature and Ca 2+ transients were recorded using a Yokagawa spinning disk confocal (491 nm excitation, 510 nm emission) with a high speed camera (Cascade 128+). For measurement of spark activity, the field stimulation was stopped and images were acquired after 2 s and analysed using Sparkmaster plugin for Image J (background fl. U: 10, criteria: 3.8, no of intervals: 1) [70] . NFκB activity assays Transgenic 6- to 8-week old male mice expressing firefly luciferase driven by two copies of the NFκB regulatory element (Jackson Laboratories Stock #006100) were swim exercised for 2 days, two sessions per day for 90 min separated by 4 h. Two hours after the final session atria and ventricles (dissected and quickly rinsed in cold PBS) were flash frozen in liquid nitrogen. Luciferase activity was assessed in tissue homogenates according to the manufacturer’s specification (Promega), and the values were standardized to total protein concentration (Bio-Rad). Statistical analysis Data are presented as mean±s.e.m.. Statistical significance was determined using unpaired or paired student’s t -test (two-tailed) as appropriate, a repeated measure one-way ANOVA with Sidak’s multiple comparison test, or a repeated measure two-way ANOVA with Sidak’s multiple comparison test. Welch’s t -test was used when the variance differed between groups (assessed via F -test). The Mann – Whitney U-test was used to compare AF durations as the data were not normally distributed according to a D’Agostino& Pearson omnibus normality test. For comparison of arrhythmic events between different treatment groups, a 2 × 2 contingency table using χ 2 -test without yates correction was used. P values <0.05 were considered statistically significant. How to cite this article: Aschar-Sobbi, R. et al . Increased atrial arrhythmia susceptibility induced by intense endurance exercise in mice requires TNFα. Nat. Commun. 6:6018 doi: 10.1038/ncomms7018 (2015). Accession codes: Microarray data have been deposited in ArrayExpress under accession code E-MTAB-3106 .